Quantum well states and amplified spin-dependent Friedel oscillations in thin films Electrons mediate many of the interactions between atoms in a solid. Their propagation in a material determines its thermal, electrical, optical, magnetic and transport properties. Therefore, the constant energy contours characterizing the electrons, in particular the Fermi surface, have a prime impact on the behaviour of materials. If anisotropic, the contours induce strong directional dependence at the nanoscale in the Friedel oscillations surrounding impurities. Here we report on giant anisotropic charge density oscillations focused along specific directions with strong spin-filtering after scattering at an oxygen impurity embedded in the surface of a ferromagnetic thin film of Fe grown on W(001). Utilizing density functional theory, we demonstrate that by changing the thickness of the Fe films, we control quantum well states confined to two dimensions that manifest as multiple flat energy contours, impinging and tuning the strength of the induced charge oscillations which allow to detect the oxygen impurity at large distances (≈50 nm). Friedel oscillations arise from the charge screening of localized defects by the electron gas of metals. The form and the magnitude of these oscillations do not depend only on the shape of the Fermi surface of the host but also on the nature of the defects. On the surface of noble metals, where the constant energy contour of the surface state is isotropic, lateral ring-like isotropic Friedel oscillations emanating from step edges and adatoms have been observed and predicted (see, for example, refs 1 , 2 , 3 , 4 , 5 , 6 ). However, if the Fermi surface is anisotropic and bears flat regions where its curvature is small or vanishes, a focusing effect with a strong directional bundling of group velocities can shape the electronic propagation at the nanoscale after scattering with defects [7] , [8] , [9] . This has been shown for Co impurities buried below copper surfaces by measurements performed with a scanning tunnelling microscope (STM) combined with density functional theory (DFT)-based simulations using the Korringa–Kohn–Rostoker Green function method [7] , [8] . As a consequence, in real, bulk materials Friedel oscillations are strongly anisotropic and can decay slower than 1/ R 3 contrary to the general wisdom stating that the confinement or dimensionality ( D ) of the electron gas defines the decay of the charge oscillations ( R − D ). It was envisioned that a quantum mechanics-induced phenomenon such as the focusing effect can be utilized in a nanosonar device that would allow to detect hidden buried impurities as well as buried nanostructures [7] . The confinement of charge density oscillations leads to quantum well states (QWS), which underlie many intriguing phenomena, such as the modulated superconducting transition temperature in thin films [10] , the quantum oscillation of surface chemical reactivities [11] , the variation of Rashba splitting in topological insulators [12] , the oscillatory interlayer exchange coupling between magnetic films across a non-magnetic spacer and the giant magnetoresistance [13] , [14] , [15] . In particular, these QWS can get spin split in noble metals on magnetic substrates [16] , [17] as measured by photoemission experiments. Similar to thin films, the charge density oscillations govern the magnetic interactions among single atoms and could act as a communication tool between nano-objects [18] , [19] , [20] , [21] . Thus, their impact in nanotechnologies is not negligible. For instance, these waves are important for the self-assembly of superstructures of adatoms on surfaces [4] , while the magnetic interactions (RKKY type) lead to unforeseen magnetic ground states [19] , [21] , [22] , [23] , [24] . Controlling and understanding the decay of these interactions, intimately related to the decay of the charge density oscillations, is decisive if these atoms are used as building blocks in nanospintronic devices. The ability to manipulate the energy contours, and in particular Fermi surfaces, with appropriate properties such as their shape and in particular their flatness, is desirable to control the magnitude of Friedel oscillations. In this work, we propose the use of exchange split QWS in magnetic thin films to design two-dimensional (2D) Fermi surfaces with multiple, film-thickness-dependent, flat energy contours leading to an extraordinarily slow lateral decay of the charge density oscillation. Depending on the quantum number defining the QWS, the spatial localization of these states changes from layer to layer. This is different from the case of a surface state which is strongly confined on the surface layer. This idea concretized after the experimental observation of unexpected anisotropic charge density oscillations around the Fermi energy due to a non-magnetic impurity, most probably oxygen, implanted in the surface of a thin Fe film grown on W(001) surface [25] . These Friedel oscillations show four-fold in-plane symmetry and are focused along the diagonal ‹110› directions of the crystal surface as observed in the d I /d U map for three monolayers (MLs) Fe on W(001) at U =−0.1 eV. Surprisingly, these oscillations extinguish if a thinner Fe film is considered, that is, two instead of three MLs. To understand this experimental result, we utilize DFT to evaluate the charge density induced by the insertion of an oxygen impurity in the ferromagnetic surface of two and three MLs Fe deposited on W(001) surface. After explaining the aforementioned experimental measurement, we assess the spin-nature of the measured Friedel oscillations and relate their focus along specific directions to the existence of QWS with flat constant energy contours that occur not only for three Fe MLs but also for thicker films. Moreover, we indicate the possible fundamental and technological implications of such lateral spin-density oscillations. 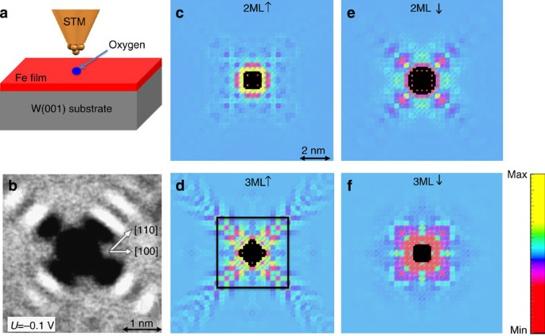Figure 1: Charge density oscillations induced around an impurity on thin Fe films on W(001). (a) STM tip scanning the Fe film surface where the oxygen impurity is implanted. The Fe film is grown on the (001) surface of W. (b) Measured charge density of states (dI/dUmap) using a W-tip at the vicinity of the Fermi energy (U=−0.1 eV) induced by an oxygen impurity on three MLs Fe/W(001) (ref.25) where the bright (dark) colour stands for charge density accumulation (depletion). Comparison with the spin-resolved theoretical charge density oscillations for states at the Fermi energy emanating from an oxygen impurity for two film thicknesses: two and three MLs for the majority-spin channel (c) and (d) followed by the corresponding ones for the minority-spin channel (e) and (f). The square indencompasses the region probed experimentally and the black spots are obtained after an uppercut of the theoretical data. Two and three MLs of Fe on W(001) Figure 1a represents a schematic of the STM measurements of the charge oscillations induced by an oxygen impurity embedded in the surface of Fe thin films on W(001) surface. The resulting highly anisotropic charge oscillations are illustrated in Fig. 1b [25] , while Fig. 1c–f illustrate the spatial modulation of the induced charge density at the Fermi energy due to the oxygen atom calculated in the vacuum at a distance of 3.165 Å above the Fe surface layer for different spin channels. Details about the theoretical methods based on DFT are given in the Methods section and Supplementary Note 1 . The Fe films are considered in their ferromagnetic ground states but we point out that contrary to 1 ML Fe/W(100) characterized by an antiferromagnetic ground state of the Fe ML [26] , [27] , thicker Fe films on the same substrate are ferromagnetic [28] . The four-fold symmetry of the anisotropic oscillations observed in the experiment is obtained theoretically and is notably pronounced for the majority-spin channel of three MLs Fe and much stronger than those of its minority-spin channel or those obtained from both spin channels of two MLs Fe. The majority-spin density oscillations in the [110] direction have the highest amplitude and survive the longest away from the impurity. These results imply spin filtering in that the spin-nature of the oscillations observed experimentally are mostly of majority-spin type. As explained below, this surprising behaviour is induced by the confinement effects in the Fe films. Figure 1: Charge density oscillations induced around an impurity on thin Fe films on W(001). ( a ) STM tip scanning the Fe film surface where the oxygen impurity is implanted. The Fe film is grown on the (001) surface of W. ( b ) Measured charge density of states (d I /d U map) using a W-tip at the vicinity of the Fermi energy ( U =−0.1 eV) induced by an oxygen impurity on three MLs Fe/W(001) (ref. 25 ) where the bright (dark) colour stands for charge density accumulation (depletion). Comparison with the spin-resolved theoretical charge density oscillations for states at the Fermi energy emanating from an oxygen impurity for two film thicknesses: two and three MLs for the majority-spin channel ( c ) and ( d ) followed by the corresponding ones for the minority-spin channel ( e ) and ( f ). The square in d encompasses the region probed experimentally and the black spots are obtained after an uppercut of the theoretical data. Full size image Quantum well states QWS of metallic films on substrates can be fully localized in the film. This naturally occurs for insulator or semiconductor substrates, since in the energy gap of the insulator there are no states available for interaction with the metallic-layer states. The states are then confined in the metallic layer, with small exponential tails in the vacuum region and in the substrate. However, localized states can also occur for metallic overlayers on metallic substrates. When the three-dimensional (3D) Fermi surface of the substrate is projected on the 2D surface Brillouin zone, there can be regions that are not covered by the projected Fermi surface. If the crystal momenta k of Bloch states with the projection k || = q of the overlayer fall in such regions, these states cannot propagate into the substrate. Then QWS, confined in the overlayer, are formed at these particular regions of the surface Brillouin zone. Practically, all metals have such a q -dependent gap region. They are rather large for the body centred cubic metals W, Mo and Cr. The projected 2D Fermi surface of W for the (001) Brillouin zone is shown in Fig. 2a . In addition to the four-fold symmetries, one sees rather large gap regions along the directions, while states exist around the origin q =0 and along the x and y axis, that is, along the directions. 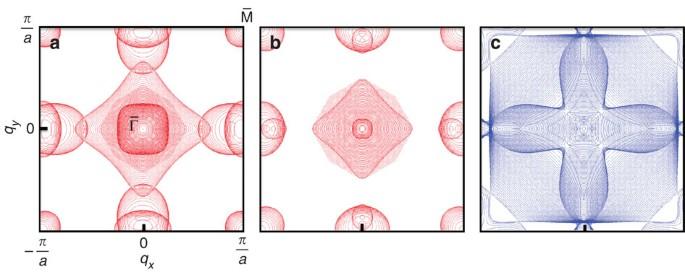Figure 2: Projected Bloch spectral function of bulk W and Fe at the Fermi energy plotted in the reciprocal space. The bulk Fermi surface is projected onto the (001) surface Brillouin zone for (a) W, (b) Fe minority-spin channel and (c) Fe majority-spin channel. Figure 2: Projected Bloch spectral function of bulk W and Fe at the Fermi energy plotted in the reciprocal space. The bulk Fermi surface is projected onto the (001) surface Brillouin zone for ( a ) W, ( b ) Fe minority-spin channel and ( c ) Fe majority-spin channel. Full size image When we compare the electronic structure of ferromagnetic Fe with the one of W (or Cr), we find that in the vicinity of E F the minority-spin Fe bands are similar to the W bands, just shifted somewhat to higher energies. Therefore, also the Fermi surface of Fe minority electrons is similar to the one of W (or Cr) and the same is true for the (001)-projected 2D Fermi surface ( Fig. 2b ). There are also rather big q -gaps along the directions and minority-spin QWS cannot occur in this q -region. However, the situation is very different for the Fe majority-spin states. There the projected Fermi surface covers nearly the whole (001) surface Brillouin zone ( Fig. 2c ). 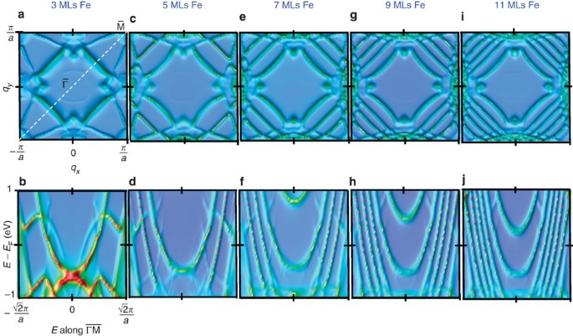Figure 3: QWS in the majority-spin channels of Fe films/W(001) surface. The upper figures exhibit the two-dimensional Bloch spectral function in the first Brillouin zone of the majority-spin channel of Fe surface atoms at the Fermi energy. Results for five different film thicknesses are depicted, that is, 3, 5, 7, 9 and 11 Fe MLs on W(001). In the lower pictures, the energy dependence of the spectral function along thedirection (dashed-line in upper left) is plotted for the respective film thicknesses. Consequently, one expects that a thicker Fe layer shows QWS confined for q -values within those gap regions of W. Figure 3 shows the appearance of such QWS with increasing layer thickness. The 2D Bloch spectral function of the Fe surface atoms at the Fermi energy is plotted in the upper figures for Fe layer thicknesses of 3, 5, 7, 9 and 11 MLs (see Supplementary Note 2 and Supplementary Fig. 1 for the case of an even number of MLs). As one sees, the gap regions are filled with an increasing number of confined states, one state for 3 MLs, two for 5 MLs and five for 11 MLs and so on. Most important is that these states show nearly no dispersion, that is, they are straight lines perpendicular to the ‹110› diagonals. Therefore, the group velocities of all these states are focused in the ‹110› directions. The lower pictures show the energy dependence of these states for q -values along , that is, along the diagonal. Figure 3: QWS in the majority-spin channels of Fe films/W(001) surface. The upper figures exhibit the two-dimensional Bloch spectral function in the first Brillouin zone of the majority-spin channel of Fe surface atoms at the Fermi energy. Results for five different film thicknesses are depicted, that is, 3, 5, 7, 9 and 11 Fe MLs on W(001). In the lower pictures, the energy dependence of the spectral function along the direction (dashed-line in upper left) is plotted for the respective film thicknesses. Full size image The majority of the states in Fig. 3 (lower panel) show a parabolic band structure. Moreover, by increasing the layer thickness by two MLs, one additional parabola is pushed down from higher energies below the Fermi level, to accommodate the additional number of electrons. For small q -values the parabolic states are damped, due to the interaction with the W-states (see Fig. 3 ). However, at the Fermi level, the q -values are larger and fall in the W gap region; thus, the states are localized. In contrast to the majority-spin channel, surface states or resonant states can occur in the minority-spin channel but disappear below the Fermi energy, where the experimental measurements are performed (see Supplementary Note 3 and Supplementary Fig. 2 ). The flat behaviour in the Fermi surface of the localized states in the surface Brillouin zone (upper panel of Fig. 3 ) can be qualitatively understood from the 3D Fermi surface of the majority-spin bands of bulk Fe. If we consider a finite, but large number N of (001) Fe layers in the vacuum, the k z -values are basically quantized into N values and the 2D Fermi surface is a projection of N slices of the 3D Fermi surface. The majority-spin Fermi surface of Fe has nearly planar areas in directions, such that the sliced Fermi surface sheets result on projection in nearly straight lines in the gap-areas. This trend can also be seen from Fig. 2c , where the 2D Fermi surface is the outcome of the projection of about 200 slices of the 3D Fermi surface. Friedel oscillations To understand the STM experiments for Fe layers on W(001), we have to discuss the Friedel oscillations around impurities in metallic systems. Using the stationary phase approximation, for large distances R from the impurities the energy-dependent charge density Δ n ( r + R ; E ) around the Fermi surface is determined from points k i on the Fermi surface, for which the group velocity v k points in the directions of R . If for a given R , only one such k -value, k 1 , exists on the constant energy surface ( E =const. ), then in three dimensions the energy-dependent charge density Δ n ( r + R ; E ) induced at a large distance R from the impurity is given by [8] where is the curvature at point k 1 measuring the flatness of the constant-energy surface, while is the component of k 1 perpendicular to the constant-energy surface. t k 1; − k 1 , δ and ϕ are energy-dependent quantities defining, respectively, the scattering strength, the phase-shift that Bloch wave functions experience after scattering and a contour-related phase. Thus, if the curvature C 1 at the surface point k 1 is small, the density change in the direction perpendicular to the constant-energy surface is particularly large resulting from the focusing of the group velocities in this direction. In fact, if C 1 vanishes, the charge density decays in this direction with a power smaller than 2. If the curvature vanishes in a region larger than a single point, then the changes are even stronger: Δ n ( r + R ; E ) decays either as 1/ R if C 1 vanishes along a line, or it does not decay at all, if C 1 vanishes in a planar area of the constant-energy surface. As discussed in ref. 8 , often more than one critical point with group velocities v k parallel to R exist, say k 1 and k 2 ; then the contributions from these two critical points are not just additive, but interfere with each other, so that three oscillation periods determined by 2 k 1 , 2 k 2 and k 1 + k 2 occur. The behaviour of Friedel oscillations in two dimensions are very similar as, for example, given by equation (1), with the modification that the amplitude decays as 1/ R only and C 1 is given by the second derivative of the constant energy line. Coming back to the calculated 2D Fermi surfaces in Fig. 3 , we can connect the QWS with the Friedel oscillation. The group velocities of all QWS point into the [110] direction, so we expect very strong charge density oscillations in these directions, as found for the three MLs case by von Bergmann et al . [25] ( Fig. 1b ) and which is in agreement with our results in Fig. 1d . Clearly only the majority-spin Fe states give rise to this, since the minority electrons do not have QWS in the gap region (see Fig. 2b ). 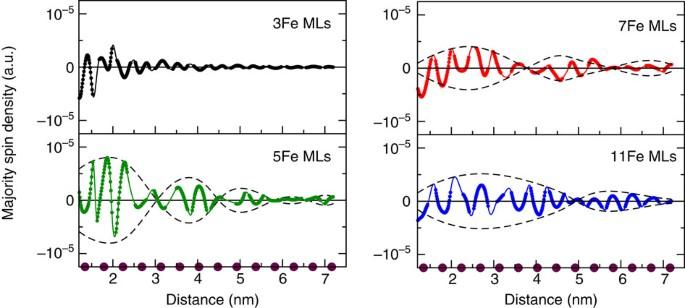Figure 4: Theoretically induced majority-spin density waves in Fe films on W(001) surface. Comparison of the majority-spin densities induced by oxygen impurity implanted in the (001) surface of Fe films with thickness of 3, 5, 7 and 11 MLs. The dashed lines are added as a guide to the eye and show different periods of higher amplitudes of the induced charge density along the surface. Figure 4 shows the calculated Friedel oscillations along the [110] direction, for 3, 5, 7 and 11 MLs of Fe. First, we see that the oscillations for three MLs are strong and very long ranged, arising from the fact that (i) the oscillations arise from a quantum well state and that (ii) the curvature of this state is very small. Moreover, due to the single QWS, the oscillations reflect the periodicity determined by the different found on parallel flat parts of the Fermi surface. The behaviour for 7 and 11 MLs shows a multiperiodicity arising from the 3 and 5, respectively, QWS. This leads to very large oscillation amplitudes, but due to partly destructive interferences this also creates an additional modulation structure with periods determined by the distance Δ k between the 3, 5, 7 and 11 different QWS. For thicker films, these nodes shift to larger distances, as one would expect from the decrease of Δ k and increase of the film thickness. In general, we expect that these oscillations, observed for three MLs Fe up to 5 nm, should be detectable for thicker films to up an order of magnitude larger distances. For two MLs, investigated experimentally [25] , the QWS does not cross the Fermi level and does not contribute to the Friedel oscillations measured at the Fermi energy. This explains the extinction of the charge ripples at large distances. Figure 4: Theoretically induced majority-spin density waves in Fe films on W(001) surface. Comparison of the majority-spin densities induced by oxygen impurity implanted in the (001) surface of Fe films with thickness of 3, 5, 7 and 11 MLs. The dashed lines are added as a guide to the eye and show different periods of higher amplitudes of the induced charge density along the surface. Full size image Concerning the minority-spin channel, we found that surface and resonant states can occur, which leads necessarily to charge oscillations. However, for three MLs, the minority-spin surface states disappear below the Fermi energy (see Supplementary Note 3 and Supplementary Fig. 2 ) and thus do not contribute to the charge density oscillations. Above the Fermi energy, oscillations are obtained but their decay is surprisingly much stronger than those obtained from the QWS of the majority-spin channel. We find large focused long-range and large amplitude majority-spin density oscillations at the Fe surface created by spin-polarized QWS of Fe films on W(100). Our finding supports the possibility to design and control of QWS in supported thin layers that lead to a super amplification of interaction effects. This may open new avenues of research by cross fertilizing communities working on QWS and on surface magnetism through the investigation of the charge or spin density oscillations along the directions parallel to the films. This can impact on the lateral coupling of magnetic nanostructures at the vicinity of the surface. For magnetic films, in particular, there is a strong amplification of a selected spin component (spin filtering), which can be detected at large distances from embedded non-magnetic defects. This may have an impact in nanotechnology, since spin information can be transmitted laterally to large distances. The choice of the substrate and the thickness of the film are of crucial importance in terms of their electronic structure to obtain a giant laterally focused signal far away from the imperfections located in the surface of thin films. Many such systems should exist, making charge density oscillations in thin films of stronger importance than in bulk materials. As substrates, the (001) surfaces of W, Cr and Mo are good choices, but also the semiconductor surfaces should be interesting candidates. For the film materials, metals with relatively flat Fermi surface parts, like ferromagnetic Fe, Co and Ni, but also Pd and Pt and even the noble metals ( http://www.hzdr.de/projects/fermisur/ ) would be potential materials to create long ranged and strongly anisotropic charge density oscillations within the film. First-principles simulations The calculations are based on DFT. First, the atomic positions of Fe atoms are relaxed using the full-potential linearized augmented plane wave (FLAPW) method within DFT as implemented in the FLEUR package ( http://www.flapw.de ) [29] . The relaxations favour inwards displacements of Fe atoms along the z axis, that is, towards the substrate. Once the positions are known (see Supplementary Note 1 and Supplementary Table 1 ), the simulations are repeated with the Korringa–Kohn–Rostoker Green function method [30] in its full-potential version considering a semi-infinite W(001). The latter allows to avoid size effects using the decimation technique [31] , [32] . Once the surface is simulated, the impurity is considered and the embedding technique based on Green functions is used to evaluate the change in the charge density at different locations. How to cite this article: Bouhassoune, M. et al . Quantum well states and amplified spin-dependent Friedel oscillations in thin films. Nat. Commun. 5:5558 doi: 10.1038/ncomms6558 (2014).